An adaptive explanation for the horse-like shape of seahorses The body shape of seahorses resembles the head and neck of horses because of their curved trunk, their ventrally bent head and their long snout. Seahorses evolved from ancestral, pipefish-like species, which have a straight body. Here, we use a biomechanical analysis and show that the seahorse's peculiar head, neck and trunk posture allows for the capture of small shrimps at larger distances from the eyes compared with pipefish. The results from the mathematical modelling were confirmed by kinematic data of prey-capturing syngnathids: compared with straight-bodied pipefish, all seahorse species studied consistently show an additional forward-reaching component in the path travelled by the mouth during their strikes at prey. This increased strike distance enlarges the volume of water they can probe for food, which is especially useful for tail-attached, sit-and-wait predators like seahorses. The biomechanics of prey capture thus provides a putative selective advantage that may explain the bending of the trunk into a horse-like shape. Seahorses are carnivorous fish that hide in strategic places along the edges of reefs or seagrass beds waiting for prey to come within striking reach [1] . Seahorses capture highly evasive prey such as small shrimp or larval fishes [1] , [2] . To do so, they make use of a two-phase prey-capture mechanism that is commonly referred to as pivot feeding [3] , [4] : a rapid upward rotation of the head is followed by suction to draw the prey into the seahorse's snout. As suction only works within a relatively short distance of the mouth [5] , [6] , bringing the mouth quickly close to the prey by rotating the head is critical to prevent prey from escaping. Syngnathid fishes (seahorses, pipefish and seadragons) are therefore equipped with large tendons of the epaxial muscles, in which they store and release elastic energy that accelerates the head towards the prey in astonishingly little time (<0.005 s) [7] , [8] . Apart from the tendons that enable extremely quick mouth displacement by cranial rotation, other unique anatomical features have evolved in syngnathid fishes [9] . The most striking feature is probably the bent position of the head relative to the trunk, which gives seahorses their horse-like appearance [10] . As a recent study showed that the Eocene ancestors of seahorses closely resemble the extant pipefish in having a trunk that is in line with the head [11] , evolution from a straight body to an S-curved body must have occurred. However, despite the prominent human fascination for seahorse anatomy, no functional explanation exists for this phenomenon. In the present study, we test whether the horse-like shape of the head and trunk of seahorses improves pivot-feeding performance. We expected the head-to-trunk position to have a biomechanical role during pivot feeding of seahorses because of an observation during previous research on the bay pipefish Syngnathus leptorhynchus [7] . In that species, a considerable ventral countermovement of the trunk occurred when the head was rotated dorsally towards the prey. This countermovement is due to the physical law of conservation of momentum. Our working hypothesis was that a trunk oriented at a sharper angle with respect to the head has an increased inertial resistance to the reaction forces of the dorsal rotation of the head, and would therefore improve head rotation performance. In other words, we expected the trunk orientation of seahorses to provide for a more stable element on which the head rotates towards the prey, compared with a pipefish-like trunk that is in line with the head, by eliminating mechanical energy wasted in ventral recoil of the trunk. We analysed both the effects of head and trunk posture on prey-capture performance via cranial rotation by using mathematical model simulations, and high-speed videos of prey capture in three seahorse species and four pipefish species. We find agreement between our model predictions and our experimental results in showing that the trajectory of the mouth depends considerably on the shape of the trunk, with a notable increase in strike distance for seahorse-like shapes. Further, we discuss the potential selective advantage of this improved aspect of prey-capture performance for seahorses in relation to their cryptic, tail-attached lifestyle. Model simulations The effect of the pipefish versus seahorse habitus on the kinematical output of cranial rotation ( Fig. 1 , Supplementary Movie 1 ) was assessed by simulating cranial rotation using two mathematical models that are basically framed on the morphology of a real pipefish and seahorse specimen ( Fig. 2 , Supplementary Movie 2 ). Gradually adjusting the head–trunk posture in each of these models allowed us to determine which aspects of cranial rotation performance are influenced by this morphological modification. We took this two-model approach because transforming the pipefish model into a more seahorse-like shape should help us to learn more about potential selective pressures or constraints acting on head–trunk morphology at the origin of the horse-like shape in the Hippocampus lineage. Similarly, modifications to the seahorse model will show us the sensitivity of seahorse performance to particular shape parameters. 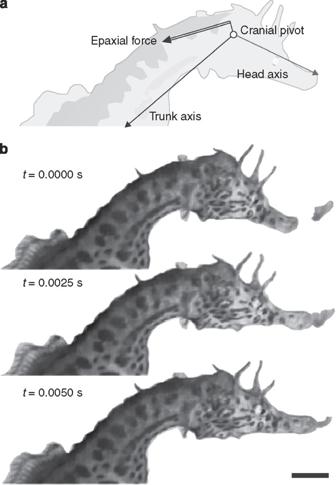Figure 1: Prey capture via cranial rotation in the seahorse. (a) Illustration of the position of the cranial joint, the head and trunk axes, and the line of action of the main force input by the epaxial muscle-tendon system. (b) Video frame sequence ofHippocampus abdominaliscapturing a mysid shrimp. Note the quick dorsal rotation of the head combined with a forward displacement of the mouth. Scale bar, 1 cm. See alsoSupplementary Movie 1. Figure 1: Prey capture via cranial rotation in the seahorse. ( a ) Illustration of the position of the cranial joint, the head and trunk axes, and the line of action of the main force input by the epaxial muscle-tendon system. ( b ) Video frame sequence of Hippocampus abdominalis capturing a mysid shrimp. Note the quick dorsal rotation of the head combined with a forward displacement of the mouth. Scale bar, 1 cm. See also Supplementary Movie 1 . 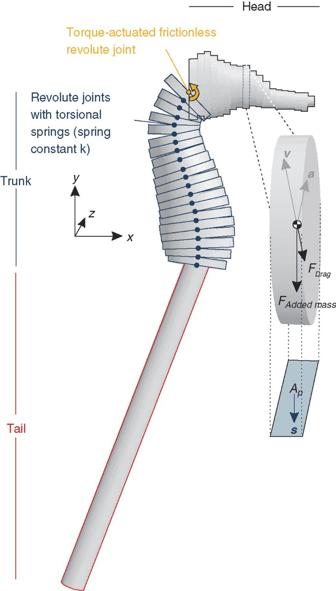Figure 2: Seahorse forward-dynamic model architecture. The external morphology is mimicked by a series of elliptical cylinders sequentially connected via joints (filled circles) that allow motion in thexyplane. Hydrodynamic resistance due to drag force (Fdrag=−0.5Cdρ Ap|v|v) and added-mass force (Fadded mass=−(a·s)sCam) are calculated for each elliptical cylinder (see enlargement). Body stiffnesskand the actuator torque profile are fine-tuned by kinematic data (see Methods for details). Symbols:a=acceleration vector,Ap=xzplane projected surface area,Ca=added mass coefficient,Cd=drag coefficient,m=elliptical cylinder mass,ρ=seawater density,s=xzsurface unit vector,v=velocity vector. See alsoSupplementary Movie 2. Full size image Figure 2: Seahorse forward-dynamic model architecture. The external morphology is mimicked by a series of elliptical cylinders sequentially connected via joints (filled circles) that allow motion in the xy plane. Hydrodynamic resistance due to drag force ( F drag =−0.5 C d ρ A p | v | v ) and added-mass force ( F added mass =−( a · s ) s C a m ) are calculated for each elliptical cylinder (see enlargement). Body stiffness k and the actuator torque profile are fine-tuned by kinematic data (see Methods for details). Symbols: a =acceleration vector, A p = xz plane projected surface area, C a =added mass coefficient, C d =drag coefficient, m =elliptical cylinder mass, ρ =seawater density, s = xz surface unit vector, v =velocity vector. See also Supplementary Movie 2 . Full size image Our mathematical model suggested that the position of the trunk relative to the head indeed had important consequences for the speed and the path of the mouth during pivot feeding in syngnathid fish ( Fig. 1 ). Forward dynamic simulations of cranial rotation revealed two main effects of sharpening the angle between the head and the trunk in the first model (based on the morphology of the pipefish S. leptorhynchus ). First, the velocity of the mouth decreased ( Fig. 3a ). Second, strike distance (defined as the distance between the starting position of the eye and the final position of the mouth) increased considerably (that is, +28%) when gradually transforming the pipefish model into a more seahorse-like shape ( Fig. 3b ). In accordance with the pipefish model results, our second model, based on the seahorse Hippocampus reidi , showed reduced velocities of the mouth travelling towards the prey (that is, −36%) compared with more elongate versions of this model ( Fig. 3c ), whereas the body shape facilitated striking at prey located a greater distance away ( Fig. 3d ). Consequently, our model highlights a trade-off between strike velocity (favoured by a head in-line with the trunk) and strike distance (favoured by sharper angles between head and trunk as observed in seahorses). Interestingly, the model predicts that this increase in strike distance is caused only by farther mouth displacement in the anterior direction (forward along the axis of the snout), and thus, not by differences in the dorsal direction in which, typically, most of the mouth motion occurs during pivot feeding in Syngathidae [3] , [7] , [12] . 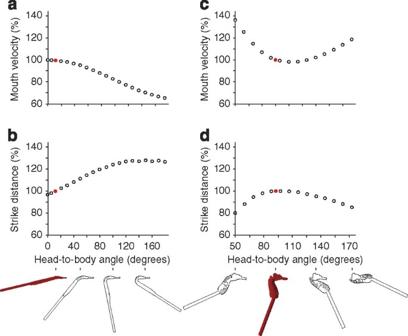Figure 3: Mathematical model simulating head rotation initiated from a range of different trunk orientations. The two feeding performance variables, mouth velocity (average instantaneous linear velocity) and strike distance (eye to prey distance), are expressed as percentages of thein vivomeasured value (indicated in red) for the pipefish model (a,b) and the seahorse model (c,d). The images below the charts illustrate the initial model geometry at four points along thexaxis. Head-to-body angle clearly has an inverse effect on the two performance traits. Note the nearly optimal anatomy of pipefish to reach the highest mouth velocity (a), and the nearly optimal position of the seahorse on the strike distance curve (d). Figure 3: Mathematical model simulating head rotation initiated from a range of different trunk orientations. The two feeding performance variables, mouth velocity (average instantaneous linear velocity) and strike distance (eye to prey distance), are expressed as percentages of the in vivo measured value (indicated in red) for the pipefish model ( a , b ) and the seahorse model ( c , d ). The images below the charts illustrate the initial model geometry at four points along the x axis. Head-to-body angle clearly has an inverse effect on the two performance traits. Note the nearly optimal anatomy of pipefish to reach the highest mouth velocity ( a ), and the nearly optimal position of the seahorse on the strike distance curve ( d ). Full size image Mouth kinematics During the strike, as predicted by our model, all seahorse species ( H. reidi , H. abdominalis , H. breviceps ) displayed movement of the mouth towards the prey with considerable anteriorly directed displacement ( Fig. 4a–c ). The pipefish species Corythoichthys intestinalis differed from the other pipefish species by behaviourally adopting a more seahorse-like, curved-trunk posture before feeding (that is, head-to-body angles larger than 20 degrees). Consequently, the path travelled by the mouth of C. intestinalis was similar to the seahorses, and a substantial forward component was measured ( Fig. 4d ). In contrast, all three straight-bodied pipefish in our sample ( Doryrhamphus melanopleura , D. dactyliophorus , S. leptorhynchus ) did not show this anterior-directed mouth displacement during feeding ( Fig. 4e–g ). Our kinematic measurements support our biomechanical model in that the path of the mouth during prey capture differs between anatomically different syngnathids, and that the mouth of species with high anterior trunk curvature can reach prey located farther away. 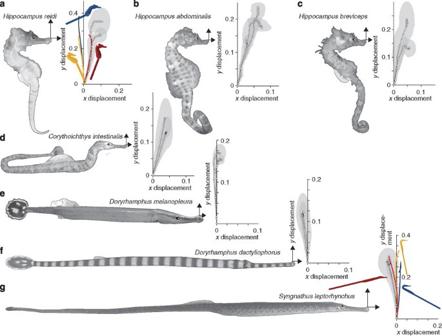Figure 4: Mouth paths during prey capture in seven species of Syngnathidae. Results are shown for the seahorsesHippocampus reidi(a),H. abdominalis(b),H. breviceps(c) and the pipefishCorythoichthys intestinalis(d),Doryrhamphus melanopleura(e),D. dactyliophorus(f) andSyngnathus leptorhynchus(g). Circles represent consecutive, averagexypositions of the snout tip expressed in fractions of head length. Left of each chart, the chart axes scaled to actual size are displayed at the snout tip of a lateral-view illustration of the species. Paths are given for two individuals per species. The grey zone surrounding each mouth path denotes the s.d. between feeding events (N=5). Mouth paths are calculated by the mathematical model ofHippocampus reidi(a) andSyngnathus leptorhynchus(g) for the original anatomy of the species (red), and the predicted effect of changes in trunk orientation (blue and yellow) are given. Figure 4: Mouth paths during prey capture in seven species of Syngnathidae. Results are shown for the seahorses Hippocampus reidi ( a ), H. abdominalis ( b ), H. breviceps ( c ) and the pipefish Corythoichthys intestinalis ( d ), Doryrhamphus melanopleura ( e ), D. dactyliophorus ( f ) and Syngnathus leptorhynchus ( g ). Circles represent consecutive, average xy positions of the snout tip expressed in fractions of head length. Left of each chart, the chart axes scaled to actual size are displayed at the snout tip of a lateral-view illustration of the species. Paths are given for two individuals per species. The grey zone surrounding each mouth path denotes the s.d. between feeding events ( N =5). Mouth paths are calculated by the mathematical model of Hippocampus reidi ( a ) and Syngnathus leptorhynchus ( g ) for the original anatomy of the species (red), and the predicted effect of changes in trunk orientation (blue and yellow) are given. Full size image If the evolution of the seahorse body shape occurred as a result of natural selection, this anatomical shift should have resulted in an increase in fitness, as might be facilitated by an increase in strike distance during feeding. As being able to strike from more distantly will increase the volume of water in which prey are susceptible to capture, the amount of potential food intake increases. In this way, the bending of the trunk into a horse-like shape, which improves the capacity to move the mouth anteriorly during the strike, can be regarded as functionally equivalent to the elongation of the snout in course of the evolution, the latter of which can be observed in several syngnathid taxa [3] , [13] . However, the true energetic and evolutionary value of increasing strike distance may depend on the foraging behaviour. Pelagic species that can efficiently chase prey would probably benefit relatively little from such changes. On the other hand, it seems logical that increasing strike distance (without decreasing strike success) is beneficial for syngnathid fishes that use a sit-and-wait strategy. The latter is indeed dominant among seahorses, which generally spend more than 80% of their time attached to the substrate or to other seahorses, during which they show slow head movements and scan the water in front of their eyes for potential prey [14] . As prehensile tail attachment is an important factor for seahorses in avoiding predators through crypsis, they seem to prefer not to swim unattached [15] . Consequently, it is likely that the differences in foraging behaviour between pipefish (which generally swim towards prey [1] , [2] ) and seahorses (which generally are tail-attached, sit-and-wait predators [15] , [16] ) may be linked to the selective pressures on either mouth velocity (evolving a pipefish-like body shape; Fig. 3a,c ) or strike distance (evolving a seahorse-like body shape; Fig. 3b,d ). Although our data cannot address this directly, the fact that the pipefish C. intestinalis was able to produce the pattern observed in seahorses ( Fig. 4 ) provides compelling support for this hypothesis, as this species is also a benthic, sit-and-wait feeder. Interestingly, it was recently suggested that the pygmy pipehorses ( Idiotropiscis ) are the sister group of Hippocampus [11] . As pygmy pipehorses have a prehensile tail but lack the bent-head posture [17] , their phylogenetic position suggests that evolution of a tail-attached lifestyle preceded the evolution of the bent head in seahorses. This provides further support for the notion that selection for increasing strike distance via increasing anterior trunk curvature arose after a sit-and-wait foraging mode has been adopted within the clade. However, as our model showed a trade-off between strike distance and mouth velocity, caused by the degree of bending of the head relative to the trunk ( Fig. 3 ), pipefish should not be regarded as inferior feeders among the extant syngnathid species. Pipefish actively locomote towards potential prey (compared with tail-attached seahorses) [1] , [2] , and thus presumably gain little to no advantage by increasing strike distance via the head alone. Moreover, a bent orientation of the head definitely increases the hydrodynamic drag during swimming [18] , which may be energetically incompatible with the more active foraging habit of a typical pipefish. The exceptional anatomy of seahorses has fascinated humans since the time of Ancient Greece (for example, Poseidon's steed), but functional explanations for this unusual body shape have not previously been proposed. Here, we suggest that the evolution from pipefish to seahorse is likely related to the biomechanics of prey capture. Because of their ventrally bent head and curved trunk, the extremely quick rotation of the head towards prey automatically results in additional anteriorly directed motion of the mouth. Therefore, rather than just serving as a more solid starting point for head rotation (our working hypothesis), the curvature in the cervical region results in a forward component of the reaction force at the neck joint in which head rotation torque is generated. This mechanical effect allows seahorses to strike at more distant prey than pipefish, which is especially useful for tail-attached, sit-and-wait predators like seahorses. Prey-capture kinematics High-speed videos (2,000 Hz) of seven species of Syngnathidae (two individuals per species) were recorded during feeding. For each individual, five prey-capture events in which the sagittal plane of the pipefish was perpendicular to the symmetry axis of the camera lens were selected. The following species (with the respective head lengths of both individuals) were obtained through aquarium trade, and were filmed with a Redlake M3 camera: C. intestinalis (12.3 and 14.7 mm), D. dactyliophorus (21.4 and 23.2 mm), D. melanopleura (9.5 and 9.8 mm), H. abdominalis (30.9 and 36.2 mm) , H. reidi (32.7 and 34.0 mm) and H. breviceps (7.8 and 8.2 mm). S. leptorhynchus (20.5 and 23.3 mm) were caught at Friday Harbor, San Juan Islands, USA and were filmed with a Redlake MotionScope camera. Animal care guidelines and regulations were strictly followed and experimental procedures were approved by the Ethical Committee of the University of Antwerp and the University of Washington Animal Care and Use Committee. For the two species that were used for biomechanical modelling ( S. leptorhynchus and H. reidi ), the kinematic profile of the head angle as well as the dorsoventral and posterior–anterior displacement of three anatomical landmarks on the anterior part of the trunk were measured. Head rotation kinematics was determined as illustrated in a previous publication [7] . The three trunk landmarks were located just posterior of the operculum, at a half head length and at a full head length along the trunk midline, and were digitized on every high-speed video frame using Didge (Alistair Cullum, Creighton University). For all species, the mouth path was determined from digitizing the upper jaw tip, and expressing the coordinates of this landmark with respect to a fixed, orthogonal frame of reference aligned with the position of the snout axis at one frame before the start of head rotation. The snout axis slope at that instant was calculated as the least-squares regression of five equally distributed landmarks digitized along the centerline of the snout. Mathematical model The head, trunk and tail were represented by a series of forty elliptical cylinders scaled to match the height and width of the head measured at specific positions on lateral and ventral view photographs ( Fig. 2 ). The head was modelled as a rigid unit of 19 elliptical cylinders connected to the body through a frictionless revolute joint (referred to as 'neck joint') allowing rotation in the dorsoventral plane. As the trunk of syngnathid fish is flexible, revolute joints with linear torsional springs were included between each of the 21 elliptical cylinders of the kinematical chain of the trunk and tail. Torque ( T ) between each two bodies, incorporated to give flexibility to the trunk, was calculated by T =− k *( α − α 0 ), were k is the spring stiffness constant, α the relative angular displacement and α 0 the spring offset of the bodies. We assumed a constant stiffness along the trunk. For each elliptical cylinder, the inertial properties and hydrodynamic resistance was accounted for ( Fig. 2 ). The model was implemented in Matlab Simulink 7.8.0 equipped with the SimMechanics 3.1 toolbox (The Mathworks). The equations of motion for this multibody system are derived automatically by SimMechanics. The equations related to hydrodynamic forces, included in the Simulink model as external forces acting on each part of the model, are illustrated in Figure 2 . The validity of these analytical, hydrodynamic equations during pivot feeding is confirmed by computational fluid dynamics [19] . The model was set in motion by a time-varying torque applied to the cranial pivot. S. leptorynchus and H. reidi served as the model species for pipefishes and seahorses, respectively. Because the motion of an open kinematic chain is simulated, differential equation solving was required. We used Matlab's inbuilt ordinary differential equation solver ODE23 (Bogacki-Shampine) with the default variable time-stepping scheme. To avoid algebraic loops, velocities and accelerations from the previous time step were used for calculating the hydrodynamic forces. Two parameters are currently still unknown for the model to be used as a forward dynamic simulation (that is, calculating motion from a given torque input): the input torque about the neck joint and the stiffness of the trunk ( k ). We determined these parameters by kinematical fine-tuning, using 2,000 Hz high-speed video data on the rotation of the head, and the dorsoventral and posterior–anterior displacement of three anatomical landmarks on the anterior part of the trunk (two individuals per species, N =5 per individual). More specifically, for four values of k , the corresponding torque profile that generated the closest match in head rotational velocity kinematics was determined iteratively. The resulting trunk kinematics ranged from too flexible (too high amplitude, too low speed of the shockwave travelling from neck joint to tail) to too stiff (too low amplitude, too high shockwave speed) compared with the in vivo anterior-trunk kinematics. The in-between value of k that showed the best match with the measured kinematics was used in the subsequent simulations with a range of different trunk orientations. In these simulations, input torque amplitude was iteratively adjusted so that the mechanical work of rotation about the neck joint remained equal. This corresponds to a situation in which always an equal amount of elastic energy is released from the head rotator tendons. How to cite this article: Van Wassenbergh, S. et al . An adaptive explanation for the horse-like shape of seahorses. Nat. Commun. 2:164 doi: 10.1038/ncomms1168 (2011).